Aberrant splicing of U12-type introns is the hallmark of ZRSR2 mutant myelodysplastic syndrome Somatic mutations in the spliceosome gene ZRSR2 —located on the X chromosome—are associated with myelodysplastic syndrome (MDS). ZRSR2 is involved in the recognition of 3′-splice site during the early stages of spliceosome assembly; however, its precise role in RNA splicing has remained unclear. Here we characterize ZRSR2 as an essential component of the minor spliceosome (U12 dependent) assembly. shRNA-mediated knockdown of ZRSR2 leads to impaired splicing of the U12-type introns and RNA-sequencing of MDS bone marrow reveals that loss of ZRSR2 activity causes increased mis-splicing. These splicing defects involve retention of the U12-type introns, while splicing of the U2-type introns remain mostly unaffected. ZRSR2-deficient cells also exhibit reduced proliferation potential and distinct alterations in myeloid and erythroid differentiation in vitro . These data identify a specific role for ZRSR2 in RNA splicing and highlight dysregulated splicing of U12-type introns as a characteristic feature of ZRSR2 mutations in MDS. Myelodysplastic syndromes (MDS) encompass a heterogeneous group of haematologic disorders collectively defined by aberrant differentiation of myeloid precursors in the bone marrow [1] , [2] . Because of the ageing of our population, the incidence of the disease is increasing rapidly [3] . MDS is characterized by accumulation of abnormal myeloid precursors in the marrow, which is accompanied by peripheral blood cytopenias. MDS often progresses to acute myeloid leukemia (AML), with a poorer prognosis compared with de novo AML [4] , [5] . Somatic mutations in several crucial genes including TET2 , DNMT3A , RUNX1 , ASXL1 and EZH2 have been implicated as causal genetic alterations in MDS [6] , [7] . More recently, second-generation sequencing of MDS identified a high frequency of somatic mutations in the genes encoding for the RNA splicing machinery [8] . Recurrent mutations were detected by us and others in SF3B1 , SRSF2 , U2AF1 , ZRSR2 and other spliceosome genes in independent cohorts of MDS, signifying a novel mechanism regulating the pathogenesis of this disease [9] , [10] , [11] , [12] , [13] , [14] . However, the functional consequence of these somatic mutations in the pathobiology of MDS remains largely unidentified. RNA splicing is a fundamental process in eukaryotes, which excises the intronic sequences from mRNA precursors to generate functional mRNA species. This function is carried out by the splicing machinery, which comprises RNA–protein complexes called small nuclear ribonucleoprotein particles (snRNP). The major splicing machinery (termed U2 spliceosome) involves 5 snRNPs (U1, U2, U4, U5 and U6), which function in concert with numerous other proteins to effect splicing of introns [15] . In addition, a second class of introns processed by a divergent spliceosome called minor (or U12) spliceosome was later identified [16] , [17] . The U12 machinery consists of U11, U12, U4atac, U6atac and U5 snRNPs, and recognizes distinct intronic splice sites [18] , [19] , [20] . The U12-type introns coexist with U2-type introns in several genes involved in essential cellular functions such as DNA replication, RNA processing, DNA repair and translation [21] . ZRSR2 (also known as URP ) is located on X chromosome (Xp22.1) and encodes for a splice factor involved in recognition of 3′-intron splice sites. It interacts with other components of the pre-spliceosome assembly including the U2AF2/U2AF1 heterodimer and SRSF2 (ref. 22 ). In vitro splicing assays suggest that ZRSR2 is required for efficient splicing of both the major and the minor class of introns [23] . In MDS, somatic mutations in ZRSR2 occur across the entire length of the transcript, which is in contrast to mutational hotspots observed in SF3B1 , SRSF2 and U2AF1 . Moreover, nonsense, splice-site and frame-shift mutations in ZRSR2 gene frequently occur in males, suggesting a loss of function. Mutations in ZRSR2 are more prevalent in MDS subtypes without ring sideroblasts and chronic myelomonocytic leukemia, and are associated with elevated percentage of bone marrow blasts and higher rate of progression to AML [8] , [13] . However, the mechanism linking ZRSR2 deficiency to pathogenesis of MDS has not been explored. In this study, we have evaluated the cellular and functional consequences of the loss of ZRSR2 in cell lines and patient samples. We show that ZRSR2 plays a pivotal role in splicing of the U12-type introns, while the U2-dependent splicing is largely unaffected. MDS bone marrow harbouring inactivating mutations in ZRSR2 exhibit overt splicing defects, primarily involving the aberrant retention of U12-type introns. Short hairpin RNA (shRNA)-mediated knockdown of ZRSR2 similarly leads to impaired splicing of U12-type introns. Knockdown of ZRSR2 also inhibits cell growth and alters the in vitro differentiation potential of haematopoietic cells. This study uncovers a specific function of ZRSR2 in RNA splicing and also suggests its role in haematopoietic development. Knockdown of ZRSR2 leads to specific splicing defects In MDS, somatic mutations in ZRSR2 are often inactivating alterations (nonsense, frame-shift and splice site mutations), which primarily affect the males, signifying its loss of function in these cases. To replicate the loss of ZRSR2, a lentiviral shRNA approach was used to stably downregulate its expression in human cells. Two shRNA vectors targeting ZRSR2 (ZRSR2 sh1 and sh2) were used to generate stable knockdown cells. These vectors resulted in efficient downregulation of ZRSR2 transcript and protein levels in 293T cells and leukemia cell lines, TF-1 and K562 ( Fig. 1a,b and Supplementary Fig. 1 ). 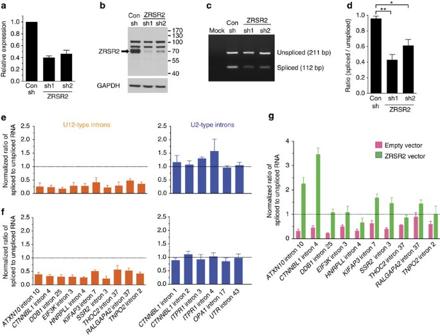Figure 1: Knockdown of ZRSR2 induces defects in splicing of U12-type introns. (a) Transcript levels ofZRSR2in TF-1 cells stably transduced with either lentiviral ZRSR2 shRNA or control (Con) vectors were examined using qRT–PCR.GAPDHlevels served as endogenous control. (b) Western blot analysis to verify the decrease in ZRSR2 protein levels in knockdown TF-1 cells. (c) Splicing efficiency of intron F ofP120minigene construct was measured in ZRSR2 knockdown and control 293T cells. A representative gel picture shows bands corresponding to unspliced and spliced product in RT–PCR analysis performed 48 h after transfection of minigene plasmid. (d) The bars depict ratio of intensities of PCR bands corresponding to spliced and unspliced products inP120minigene assay. The data represent the mean±s.e.m. of three independent transfection experiments. *P<0.05, **P<0.01; unpairedt-test. (e,f) Average ratio of spliced to unspliced pre-mRNA levels of ten U12-type and six U2-type introns in TF-1 cells on knockdown of ZRSR2 using two shRNA vectors, ZRSR2 sh1 (e) and ZRSR2 sh2 (f). The data are mean±s.e.m. from at least three independent RNA preparations. Horizontal dotted lines represent the ratio for control transduced cells, which were set as 1.0.GAPDHwas used as endogenous control. (g) Average ratios of spliced to unspliced levels of U12-type introns on transient transfection of ZRSR2 expression plasmid in knockdown 293T cells are depicted. 293T cells stably expressing ZRSR2 sh1 or control vector were transfected with either pCDNA3-hZRSR2 or empty vector, and total RNA was extracted after 72 h. The splicing efficiency was measured using qPCR and spliced/unspliced ratio was set as 1.0 for control cells transfected with empty vector (horizontal dotted line).GAPDHwas used to normalize for cDNA input. The results are average of five to seven transfection experiments and are represented as mean±s.e.m. Figure 1: Knockdown of ZRSR2 induces defects in splicing of U12-type introns. ( a ) Transcript levels of ZRSR2 in TF-1 cells stably transduced with either lentiviral ZRSR2 shRNA or control (Con) vectors were examined using qRT–PCR. GAPDH levels served as endogenous control. ( b ) Western blot analysis to verify the decrease in ZRSR2 protein levels in knockdown TF-1 cells. ( c ) Splicing efficiency of intron F of P120 minigene construct was measured in ZRSR2 knockdown and control 293T cells. A representative gel picture shows bands corresponding to unspliced and spliced product in RT–PCR analysis performed 48 h after transfection of minigene plasmid. ( d ) The bars depict ratio of intensities of PCR bands corresponding to spliced and unspliced products in P120 minigene assay. The data represent the mean±s.e.m. of three independent transfection experiments. * P <0.05, ** P <0.01; unpaired t -test. ( e , f ) Average ratio of spliced to unspliced pre-mRNA levels of ten U12-type and six U2-type introns in TF-1 cells on knockdown of ZRSR2 using two shRNA vectors, ZRSR2 sh1 ( e ) and ZRSR2 sh2 ( f ). The data are mean±s.e.m. from at least three independent RNA preparations. Horizontal dotted lines represent the ratio for control transduced cells, which were set as 1.0. GAPDH was used as endogenous control. ( g ) Average ratios of spliced to unspliced levels of U12-type introns on transient transfection of ZRSR2 expression plasmid in knockdown 293T cells are depicted. 293T cells stably expressing ZRSR2 sh1 or control vector were transfected with either pCDNA3-hZRSR2 or empty vector, and total RNA was extracted after 72 h. The splicing efficiency was measured using qPCR and spliced/unspliced ratio was set as 1.0 for control cells transfected with empty vector (horizontal dotted line). GAPDH was used to normalize for cDNA input. The results are average of five to seven transfection experiments and are represented as mean±s.e.m. Full size image First, we examined the effect of ZRSR2 deficiency on splicing, by transfection of minigene constructs in ZRSR2 knockdown and control-transduced 293T cells. Two reporter constructs commonly used to assess splicing— P120 minigene [24] and GH1 reporter plasmid [25] —were used in these experiments. P120 minigene reporter consists of exons 5–8 of human NOP2 (also known as NOL1 or P120 ) gene. We observed that the splicing of intron F, a U12-type intron, was reduced on downregulation of ZRSR2 using both ZRSR2 shRNA vectors ( Fig. 1c,d ). The GH1 minigene reporter consists of three exons, and on transfection a fully spliced and exon-skipped (missing the second exon) mRNA can be detected. Notably, in a previous study, ectopic expression of mutant U2AF1—a splice factor related to ZRSR2 and also frequently mutated in MDS—results in higher frequency of exon skipping from GH1 minigene construct [12] . We observed that ZRSR2 knockdown and control 293T cells exhibited comparable rates of exon skipping on transfection of GH1 reporter construct ( Supplementary Fig. 2 ). Therefore, our results highlight that ZRSR2 functions in a manner distinctive of U2AF1. Next, we assessed splicing of endogenous introns in the MDS/AML cell line, TF-1 (ref. 26 ), transduced with either ZRSR2 shRNA or control vector. ZRSR2 has been proposed to be involved in splicing of both major and minor classes of introns [23] ; therefore, splicing of both these types of introns was examined. All tested U12-dependent introns were less efficiently spliced in the ZRSR2 knockdown cells ( Fig. 1e,f ). The average ratio of spliced/unspliced RNA for the ten U12-type introns was 0.30 in sh1-transduced and 0.38 in sh2-transduced cells as compared with 1.0 in the control cells. Notably, the splicing of six U2-type introns was not significantly affected (spliced/unspliced ratio of 1.19 for sh1 and 0.96 for sh2 as compared with 1.0 for cells transduced with control shRNA; Fig. 1e,f ). Hence, the inability of ZRSR2 knockdown cells to splice efficiently endogenous and exogenous U12-type introns points towards a specific defect in the minor splicing machinery. To test whether overexpression of ZRSR2 can rescue the U12 splicing defects, we transiently transfected wild-type (WT) ZRSR2 into stably knock down 293T cells ( Supplementary Fig. 3a ) and measured the splicing efficiency of U12-type introns. Ectopic expression of ZRSR2 resulted in a significant increase in the splicing efficiency of all U12-type introns tested as compared with cells transfected with empty vector ( Fig. 1g and Supplementary Fig. 3b ). Therefore, we conclude that aberrant splicing observed in knockdown cells was a consequence of downregulation of ZRSR2. Overall, our experiments to evaluate splicing of endogenous and exogenous introns in ZRSR2 knockdown cells recognize its role in the U12-dependent spliceosome. Inactivating ZRSR2 mutations in MDS cause splicing defects To address the consequences of ZRSR2 mutations in MDS, a global evaluation of splicing alterations was performed using RNA sequencing (RNA-Seq). RNA was extracted from the bone marrow of eight male MDS patients harbouring either nonsense or frame-shift mutations of ZRSR2 ( Fig. 2a ) (hereafter referred to as ‘ ZRSR2 mutant MDS’). We also sequenced RNA from four MDS cases without mutation in either ZRSR2 or other commonly mutated splice factors ( U2AF1 , SF3B1 and SRSF2 ; termed ‘ ZRSR2 WT MDS’). In addition, three non-malignant bone marrows and one remission bone marrow (remission of sample 7; ZRSR2 mutant MDS; Table 1 ) were also included as controls (termed ‘normal bone marrow (BM)’). RNA-Seq verified the presence of mutations in ZRSR2 with a high mutant allele frequency (range: 67.9–98.0%) in all the ZRSR2 mutant MDS samples ( Supplementary Fig. 4 ). 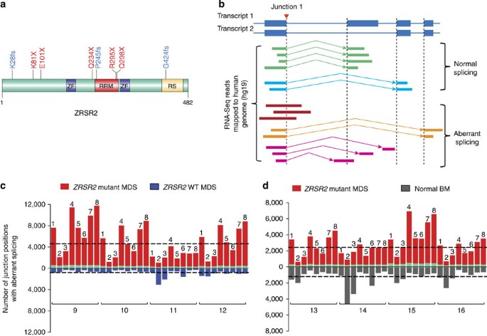Figure 2: RNA-Seq of MDS bone marrow harbouring mutations inZRSR2reveals splicing defects. (a) Schematic representation of human ZRSR2 protein with position and type of mutations in eight MDS patients used for RNA-Seq. (b) Approach used to define the RNA-Seq reads for analysis of splice junctions is shown. All splice junctions corresponding to known RefSeq transcripts were examined. Reads mapped to a representative splice position (Junction 1) are classified as either ‘normal’ or ‘aberrant’ in the illustration. (c) Number of junction positions with aberrant reads obtained in pairwise comparisons betweenZRSR2mutant and WT MDS are depicted. Junctions with significant aberrant reads inZRSR2mutant (ΔMSI >20) are shown as red bars, while those inZRSR2WT (ΔMSI <−20) are shown as blue bars for each mutant versus WT pair. The dashed horizontal lines denote the averages of aberrant junction positions in the two genotypes across 32 comparison pairs (8ZRSR2mutant MDS compared individually with 4ZRSR2WT MDS). (d) Number of aberrant junctions obtained in pairwise comparisons betweenZRSR2mutant MDS and normal BM analysed and depicted as described inc. The black bars represent number of aberrant junctions detected in normal BM. The green bars incanddrepresent the number of junctions that were identified in all eight mutant/eight control samples in at least one pairwise comparison. Each pair of bars incanddis labelled with identifiers forZRSR2mutant and control samples represented in their pair-wise comparison. The sample information including details ofZRSR2mutations are described inTable 1. Figure 2: RNA-Seq of MDS bone marrow harbouring mutations in ZRSR2 reveals splicing defects. ( a ) Schematic representation of human ZRSR2 protein with position and type of mutations in eight MDS patients used for RNA-Seq. ( b ) Approach used to define the RNA-Seq reads for analysis of splice junctions is shown. All splice junctions corresponding to known RefSeq transcripts were examined. Reads mapped to a representative splice position (Junction 1) are classified as either ‘normal’ or ‘aberrant’ in the illustration. ( c ) Number of junction positions with aberrant reads obtained in pairwise comparisons between ZRSR2 mutant and WT MDS are depicted. Junctions with significant aberrant reads in ZRSR2 mutant (ΔMSI >20) are shown as red bars, while those in ZRSR2 WT (ΔMSI <−20) are shown as blue bars for each mutant versus WT pair. The dashed horizontal lines denote the averages of aberrant junction positions in the two genotypes across 32 comparison pairs (8 ZRSR2 mutant MDS compared individually with 4 ZRSR2 WT MDS). ( d ) Number of aberrant junctions obtained in pairwise comparisons between ZRSR2 mutant MDS and normal BM analysed and depicted as described in c . The black bars represent number of aberrant junctions detected in normal BM. The green bars in c and d represent the number of junctions that were identified in all eight mutant/eight control samples in at least one pairwise comparison. Each pair of bars in c and d is labelled with identifiers for ZRSR2 mutant and control samples represented in their pair-wise comparison. The sample information including details of ZRSR2 mutations are described in Table 1 . Full size image Table 1 Details of human bone marrow samples used for RNA-Seq. Full size table First, the RNA-Seq data were examined for abnormal sequencing reads at all splice junctions to assess the extent of mis-spliced events in different groups. The ‘normal’ reads comprised those which aligned to the known exon–exon junctions, while ‘abnormal’ reads either spanned exon–intron junctions or corresponded to splicing involving an ambiguous splice site as illustrated in Fig. 2b . We examined 298,275 unique splice junctions (23,786 RefSeq transcripts in 15,737 genes) for aberrant splicing and each ZRSR2 mutant MDS sample was compared with a control sample ( ZRSR2 WT MDS or normal BM) as described in the Methods section. Using a false discovery rate (FDR) cutoff of 0.01 and difference in Mis-splicing Index (ΔMSI) >20, significantly higher number of abnormally spliced junctions were detected in ZRSR2 mutant MDS samples compared with the ZRSR2 WT MDS samples in a majority of pairwise comparisons ( Fig. 2c ). Similarly, the number of such abnormal junctions was also elevated in ZRSR2 mutant group when compared with four normal BM samples ( Fig. 2d ). These findings suggested a higher incidence of aberrant splicing in samples with ZRSR2 mutation as compared with controls. Notably, 689 mis-spliced junctions were identified in all eight ZRSR2 mutant MDS cases, signifying a subset of introns that represent bona-fide downstream targets of ZRSR2. Aberrant intron retention in ZRSR2 mutant MDS To delineate the splicing defects that occur in ZRSR2 -mutated cells, we carefully evaluated the RNA-Seq data of mutant and control bone marrows for aberrant intron retention, cryptic splice site usage and exon skipping. For identification of aberrant retention, introns with ≥95% coverage and with sequencing reads supporting both 5′ and 3′ exon–intron junctions were considered (described in Methods section). We compared the proportion of aberrant reads (spanning across both exon–intron junctions) in each sample to calculate the MSI ( Supplementary Fig. 5 ). The difference in the MSI values between the mutant and control samples (termed ΔMSI) was used as a measure of aberrant retention for each intron. Using this approach, we tested 110,192 introns and performed pairwise analyses between 8 ZRSR2 mutant MDS samples and 8 controls (4 ZRSR2 WT MDS and 4 normal BM samples) to obtain 64 sets of comparisons. We observed that elevated number of retained introns was clearly evident in ZRSR2 mutant MDS as compared with either ZRSR2 WT MDS or normal BM samples ( Fig. 3a,b ). Importantly, significant intron retention was not detected when comparing the ZRSR2 WT MDS with normal BM samples ( Fig. 3c ), underlining that the intron retention is specific to mutations in the ZRSR2 gene. 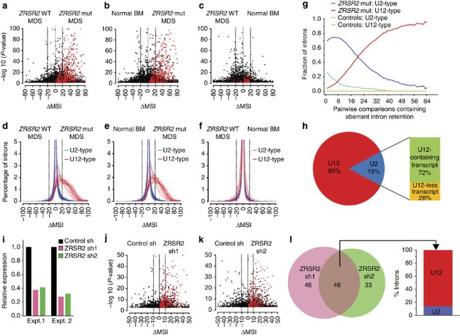Figure 3:ZRSR2-mutated MDS bone marrow and ZRSR2 knockdown cells are characterized by aberrant retention of U12-type introns. (a–c) Dot plots display aberrantly retained introns in a representative pairwise analysis ofZRSR2mutant MDS versusZRSR2WT MDS (a),ZRSR2mutant MDS versus normal BM (b), and normal BM versusZRSR2WT MDS (c). Each dot denotes an intron and U12-type introns are shown in red.P-value was calculated using Fisher’s exact test and data points withP<0.01 are shown. (d–f) Histograms depict frequencies of U2-type and U12-type introns plotted against ΔMSI values in pairwise comparisons ofZRSR2mutant and control samples. Each curve represents a pairwise comparison for U2-type (blue) and U12-type (red) intron. Thirty-two comparisons betweenZRSR2mutant MDS andZRSR2WT MDS (d), 32 comparisons betweenZRSR2mutant MDS and normal BM (e), and 16 comparisons betweenZRSR2WT MDS and normal BM (f) were performed. (g) The proportion of U2-type and U12-type introns among aberrantly retained introns in eitherZRSR2mutant or controls (ZRSR2WT MDS+normal BM) are shown for 64 pairwise comparisons. The number of introns is plotted against the number of pairwise comparisons in which they were identified. (h) Distribution of intron type for significantly retained introns (ΔMSI >20; FDR ≤0.01) inZRSR2mutant MDS is shown. The bar graph shows the distribution of retained U2-type introns into those present in either transcript containing a U12-type intron or without U12-type intron. (i) Relative expression ofZRSR2was computed as fragments per kilobase of transcript per million fragments mapped (FPKM) values from RNA-Seq data in two independently transduced control and knockdown TF-1 cells. (j,k) Dot plots depict aberrantly retained introns in control versus ZRSR2 sh1 (j) and control versus ZRSR2 sh2 (k). Only data points corresponding toP<0.01 are displayed. (l) Venn diagram shows an overlap of retained introns between ZRSR2 sh1 and sh2 knockdown TF-1 cells. The introns that are significantly retained (P<0.01; ΔMSI >10) for sh1- or sh2-transduced cells in both experiments are included. The bar graph on the right depicts the proportion of U2-type and U12-type introns among the introns retained in both sh1- and sh2-transduced cells. Figure 3: ZRSR2 -mutated MDS bone marrow and ZRSR2 knockdown cells are characterized by aberrant retention of U12-type introns. ( a – c ) Dot plots display aberrantly retained introns in a representative pairwise analysis of ZRSR2 mutant MDS versus ZRSR2 WT MDS ( a ), ZRSR2 mutant MDS versus normal BM ( b ), and normal BM versus ZRSR2 WT MDS ( c ). Each dot denotes an intron and U12-type introns are shown in red. P -value was calculated using Fisher’s exact test and data points with P <0.01 are shown. ( d – f ) Histograms depict frequencies of U2-type and U12-type introns plotted against ΔMSI values in pairwise comparisons of ZRSR2 mutant and control samples. Each curve represents a pairwise comparison for U2-type (blue) and U12-type (red) intron. Thirty-two comparisons between ZRSR2 mutant MDS and ZRSR2 WT MDS ( d ), 32 comparisons between ZRSR2 mutant MDS and normal BM ( e ), and 16 comparisons between ZRSR2 WT MDS and normal BM ( f ) were performed. ( g ) The proportion of U2-type and U12-type introns among aberrantly retained introns in either ZRSR2 mutant or controls ( ZRSR2 WT MDS+normal BM) are shown for 64 pairwise comparisons. The number of introns is plotted against the number of pairwise comparisons in which they were identified. ( h ) Distribution of intron type for significantly retained introns (ΔMSI >20; FDR ≤0.01) in ZRSR2 mutant MDS is shown. The bar graph shows the distribution of retained U2-type introns into those present in either transcript containing a U12-type intron or without U12-type intron. ( i ) Relative expression of ZRSR2 was computed as fragments per kilobase of transcript per million fragments mapped (FPKM) values from RNA-Seq data in two independently transduced control and knockdown TF-1 cells. ( j , k ) Dot plots depict aberrantly retained introns in control versus ZRSR2 sh1 ( j ) and control versus ZRSR2 sh2 ( k ). Only data points corresponding to P <0.01 are displayed. ( l ) Venn diagram shows an overlap of retained introns between ZRSR2 sh1 and sh2 knockdown TF-1 cells. The introns that are significantly retained ( P <0.01; ΔMSI >10) for sh1- or sh2-transduced cells in both experiments are included. The bar graph on the right depicts the proportion of U2-type and U12-type introns among the introns retained in both sh1- and sh2-transduced cells. Full size image We further examined the retained introns in ZRSR2 -mutated cases for the type of intron. The introns were categorized as either U2- or U12-type based on the divergence at the 5′- and 3′-splice sites and the branchpoint sequence [20] , [21] , using the computational method described previously [27] . This analysis revealed a striking overabundance of U12-type introns among the aberrantly retained introns in ZRSR2 mutant MDS samples ( Fig. 3a,b,d,e ). This pattern was observed consistently across all the pairwise comparisons between ZRSR2 mutant and control samples ( Fig. 3d,e ), while the comparisons between ZRSR2 WT MDS and normal BM (16 pairwise comparisons) did not show any intron type-specific retention ( Fig. 3f ). Next, to ascertain the subset of introns, which were consistently retained in ZRSR2 mutant samples (ΔMSI >20), we focused on introns recognized in a large number of pairwise comparisons. Expectedly, the number of aberrantly retained introns identified in successively increasing numbers of pairwise comparisons gradually decreased ( Supplementary Fig. 6 ); however, the proportion of U12-type introns among the retained introns steadily climbed ( Fig. 3g ). In fact, 43 out of 45 introns retained in the ZRSR2 mutant MDS in all 64 comparisons were U12 dependent. On the other hand, specific intron retention in the ZRSR2 WT and normal BM groups (ΔMSI <−20) was not apparent and no intron was retained in more than 41 pairwise comparisons ( Fig. 3g ). Consequently, among the high-ranking set of introns consistently retained (present in >41 pairwise comparisons) in the ZRSR2 mutant MDS, a disproportionately higher prevalence (85%) of U12-type introns occurred ( Fig. 3h and Supplementary Data 1 ), thereby underscoring the involvement of ZRSR2 in the minor spliceosome machinery. Moreover, among the retained U2-type introns, 72% were contained in a transcript also harbouring a U12-type intron, with the retained U2-type intron typically located immediately downstream of the U12-type intron ( Fig. 3h and Supplementary Fig. 7 ). This indicates that the inefficient splicing of U12-type introns can also cause mis-splicing of neighbouring U2-type introns within the transcript. Only 11 U2-type introns, which were independent of U12 transcripts, were identified as aberrantly retained in our computational approach ( Supplementary Data 1 ). These introns were indistinguishable from other unaffected U2-type introns (data not shown) and invariably displayed a weaker retention phenotype compared with the U12-type introns. Although our preceding analysis identified that the U12-type introns were significantly retained in ZRSR2 mutant MDS, we further inquired whether the splicing of all U12-type was affected. To address this, we examined the aberrant retention of each U12-type intron using the average ΔMSI values for mutant versus control groups. Of all the genes harbouring U12-type introns in the human genome [27] , [28] , genes containing 558 U12 introns were expressed at sufficient levels (FPKM max >1; FPKM average >0.5). First, ΔMSI calculations showed that practically all U12-type introns were mis-spliced, albeit to varying extent, in the ZRSR2 mutant MDS group ( Supplementary Fig. 8 ). This is also evident in individual pairwise comparisons between ZRSR2 mutant MDS and control samples ( Fig. 3d,e ). Next, we classified the U12-type introns based on the ΔMSI values and found that the splicing of only 29 introns (ΔMSI ≤0) (5% of expressed U12-type introns) was unaffected ( Supplementary Data 2 ). Although, we did not detect any difference in the distribution of GT-AG versus AT-AC intron type with the retention phenotype, the U12-type introns, which are not retained in ZRSR2 mutant cells, tend to be longer (median length 1,958 nucleotides compared with 1,039 for significantly retained introns; Supplementary Data 2 ). Interestingly, the unaffected GT-AG introns had relatively weaker splice sites as indicated by lower 5′-splice site score compared with the retained introns ( Supplementary Data 2 ). We also sequenced mRNA from TF-1 cells in which ZRSR2 was downregulated, using either sh1 or sh2 lentiviral vectors. Stable knockdown cells from two independent transduction experiments were used to examine for intron retention as described above. Expression analysis confirmed 60–70% reduction in ZRSR2 transcript levels in the knockdown cells ( Fig. 3i ). The suppression of ZRSR2 in these knockdown cells resulted in marked retention of U12-type introns as compared with control shRNA-transduced cells ( Fig. 3j,k ). Overall, the number of retained introns obtained in knockdown TF-1 cells was lower than those identified in ZRSR2 mutant MDS cases. This is conceivable because of low levels of ZRSR2 present in the knockdown cells as compared with complete absence in males with either nonsense or frame-shift mutations. Importantly, among the introns retained in both sh1 and sh2 knockdown cells, a large proportion were U12-type introns ( Fig. 3l ). Notably, we observed a sizeable overlap of U12-type introns retained in both ZRSR2 mutant MDS and knockdown TF1 cells ( Supplementary Fig. 9 ). Next, to validate the aberrant intron retention, quantitative reverse transcriptase–PCR (qRT–PCR) was used to measure the normalized intronic expression in ZRSR2 mutant MDS and control samples. Using this approach, we tested eight representative U12-type introns detected as aberrantly retained in our computational analysis. We observed markedly higher expression of all tested introns in each of the mutant samples as compared with the control samples ( Fig. 4a–h ). In a parallel analysis, we also detected higher expression of these introns in ZRSR2 knockdown TF1 cells ( Supplementary Fig. 10 ), signifying consistent findings in our two experimental models. 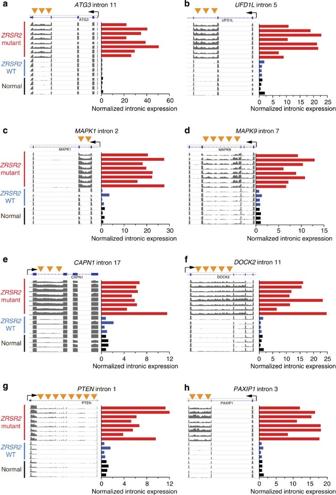Figure 4: Detection of U12-type intron retention inZRSR2mutant MDS. (a–h) Normalized intron expression for eight representative U12-type introns was determined using qPCR. The RNA-Seq reads normalized to total number of mappable reads for all 16 cases are depicted using IGV 2.3 in the left panels. Read counts are shown using an identical scale in all samples, and the U12-type introns are indicated by orange arrow heads. For each gene, only the genomic locus containing the retained intron is shown. Right panels: the expression of U12-type introns was measured relative to the expression of flanking exons and is shown by horizontal bars (red bars,ZRSR2mutant MDS; blue bars,ZRSR2WT MDS; black bars, normal BM). Figure 4: Detection of U12-type intron retention in ZRSR2 mutant MDS. ( a – h ) Normalized intron expression for eight representative U12-type introns was determined using qPCR. The RNA-Seq reads normalized to total number of mappable reads for all 16 cases are depicted using IGV 2.3 in the left panels. Read counts are shown using an identical scale in all samples, and the U12-type introns are indicated by orange arrow heads. For each gene, only the genomic locus containing the retained intron is shown. Right panels: the expression of U12-type introns was measured relative to the expression of flanking exons and is shown by horizontal bars (red bars, ZRSR2 mutant MDS; blue bars, ZRSR2 WT MDS; black bars, normal BM). Full size image The experimental evidence of U12-type intron retention specifically in ZRSR2-deficient MDS samples further substantiates ZRSR2 as a crucial component of the U12-dependent spliceosome. Additional mis-splicing events in ZRSR2 mutant MDS Further, using an approach similar to the one to detect intron retention, we searched for mis-splicing events involving abnormal recognition of 5′- and 3′-splice sites ( Supplementary Fig. 5 ). We identified several loci where cryptic splice sites were observed in ZRSR2 mutant MDS. We focused on loci, which displayed aberrant splicing in all mutant cases, and found that the majority of them were associated with transcripts containing U12-type introns. These events usually occurred either within the U12-type introns or in their vicinity. The incorrect recognition of splice sites resulted in a varied pattern of mis-splicing involving ambiguous splice donor and acceptor sites, which invariably generated cryptic U2 splice junctions ( Fig. 5 ). As representative examples of abnormal splice site recognition in ZRSR2 mutant MDS, mis-spliced U12-type introns in WDR41 , FRA10AC1 and SRPK2 genes were experimentally validated. 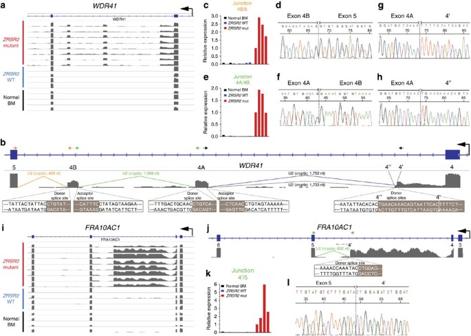Figure 5: Cryptic splice junctions in U12-type introns ofWDR41andFRA10AC1. (a) Normalized RNA-Seq reads mapped to the genomic region encompassing exons 4 and 5 ofWDR41gene are displayed using IGV 2.3 for all 16 samples. Reads in all samples are shown on identical scale. (b) Aberrant splice junctions in intron 4 (U12-type intron) ofWDR41gene are depicted. The mis-spliced regions (designated 4A and 4B) and two alternative splice donor sites in intron 4 (upstream of 4A; marked as 4’ and 4’’) inZRSR2mutant samples are illustrated. The intron type and length for the cryptic junctions are indicated. The cryptic splice acceptor and donor sequences, which are activated inZRSR2mutant MDS, are shown below. The PCR primers used incandeare indicated by arrows. (c,d) Experimental verification of splicing junction between 4B and exon 5 ofWDR41. (c) qRT–PCR using primers located in 4B and exon 5 to determine relative levels of mis-spliced transcript inZRSR2mutant and control samples. (d) The PCR product amplified from cDNA ofZRSR2mutant samples incwas Sanger sequenced. The junction is shown by dashed vertical line. (e,f) Splicing between 4A and 4B was analysed as described above incandd, respectively. (g,h) Sanger sequencing of the PCR amplicon obtained from cDNA ofZRSR2mutant samples using primers located in 4A and retained intron (upstream of 4′). The PCR product was cloned into TOPO TA vector and individual clones were sequenced to verify two alternative splice donor sites (4′ and 4″). (i) RNA-Seq reads mapped to the genomic region encompassing exons 3–6 ofFRA10AC1gene. (j) Aberrant splice donor site (denoted 4′) in intron 4 ofFRA10AC1is shown for a representativeZRSR2mutant sample. Sequence and intron-type for the cryptic splice junction are indicated. (k) qRT–PCR to measure the relative levels of mis-spliced RNA inZRSR2mutant and control samples using primers located in intron 4 and exon 5.GAPDHwas used to normalize the levels of transcripts. (l) Sanger sequencing of the PCR product obtained fromZRSR2mutant samples inj. The junction between intron 4 and exon 5 is indicated by the dashed vertical line. Figure 5: Cryptic splice junctions in U12-type introns of WDR41 and FRA10AC1 . ( a ) Normalized RNA-Seq reads mapped to the genomic region encompassing exons 4 and 5 of WDR41 gene are displayed using IGV 2.3 for all 16 samples. Reads in all samples are shown on identical scale. ( b ) Aberrant splice junctions in intron 4 (U12-type intron) of WDR41 gene are depicted. The mis-spliced regions (designated 4A and 4B) and two alternative splice donor sites in intron 4 (upstream of 4A; marked as 4’ and 4’’) in ZRSR2 mutant samples are illustrated. The intron type and length for the cryptic junctions are indicated. The cryptic splice acceptor and donor sequences, which are activated in ZRSR2 mutant MDS, are shown below. The PCR primers used in c and e are indicated by arrows. ( c , d ) Experimental verification of splicing junction between 4B and exon 5 of WDR41 . ( c ) qRT–PCR using primers located in 4B and exon 5 to determine relative levels of mis-spliced transcript in ZRSR2 mutant and control samples. ( d ) The PCR product amplified from cDNA of ZRSR2 mutant samples in c was Sanger sequenced. The junction is shown by dashed vertical line. ( e , f ) Splicing between 4A and 4B was analysed as described above in c and d , respectively. ( g , h ) Sanger sequencing of the PCR amplicon obtained from cDNA of ZRSR2 mutant samples using primers located in 4A and retained intron (upstream of 4′). The PCR product was cloned into TOPO TA vector and individual clones were sequenced to verify two alternative splice donor sites (4′ and 4″). ( i ) RNA-Seq reads mapped to the genomic region encompassing exons 3–6 of FRA10AC1 gene. ( j ) Aberrant splice donor site (denoted 4′) in intron 4 of FRA10AC1 is shown for a representative ZRSR2 mutant sample. Sequence and intron-type for the cryptic splice junction are indicated. ( k ) qRT–PCR to measure the relative levels of mis-spliced RNA in ZRSR2 mutant and control samples using primers located in intron 4 and exon 5. GAPDH was used to normalize the levels of transcripts. ( l ) Sanger sequencing of the PCR product obtained from ZRSR2 mutant samples in j . The junction between intron 4 and exon 5 is indicated by the dashed vertical line. Full size image The intron 4 of human WDR41 gene is a U12-type intron. RNA-Seq revealed a distinctive pattern of mis-splicing in all ZRSR2 mutant samples, which includes retention of the 5′-portion of the intron followed by multiple mis-splicing events employing cryptic U2-type splice sites within intron 4 ( Fig. 5a,b and Supplementary Data 3 and 4 ). We verified the presence of such aberrant splice junctions across the exons 4 and 5 involving two cryptic exons (‘4A’ and ‘4B’) using qRT–PCR. The levels of mis-spliced products were substantially higher in the ZRSR2 mutant MDS as compared with either the ZRSR2 WT MDS or normal BM samples ( Fig. 5c,e ). Moreover, Sanger sequencing of the products amplified from ZRSR2 mutant samples verified the predicted splice junctions ( Fig. 5d,f ). We detected two alternative splice donor sites (4′ and 4″ located 19 bp apart) both of which resulted in splicing to cryptic exon 4A ( Fig. 5g,h ). Similarly, in FRA10AC1 and SRPK2 , anomalous splice junctions were created from cryptic U2-type splice sites, which resulted in partial retention of U12-type introns in ZRSR2 mutant samples ( Fig. 5i,j , Supplementary Fig. 11a,b and Supplementary Data 3 and 4 ). The presence of these alternative splicing junctions was also validated by PCR and Sanger sequencing ( Fig. 5k,l and Supplementary Fig. 11c,d ). Likewise, in conventional RT–PCR analysis of WDR41 , FRA10AC1 and SRPK2 , aberrantly spliced transcripts were detectable only in ZRSR2 mutant MDS samples ( Supplementary Fig. 12 ). We also detected a few instances of increased exon skipping in the ZRSR2 mutant group. The exon skipping phenotype was observed in the transcripts containing the U12-type introns and often involved exons flanking the U12-type intron ( Supplementary Data 5 ). Downregulation of ZRSR2 alters growth and differentiation We investigated the consequences of ZRSR2 suppression on cell growth and haematopoietic differentiation, using shRNA-mediated knockdown. We observed that the ZRSR2-deficient leukemia cells divided moderately slower than the cells transduced with control shRNA vector (data not shown). In soft agar colony assay, downregulation of ZRSR2 resulted in pronounced reduction in the number of colonies obtained in TF-1 and K562 cells ( Fig. 6a ). In propidium iodide staining of steady-state TF-1 cells, fewer cells were detected in S-phase of the cell cycle ( Supplementary Fig. 13a ). In addition, lower proportion of ZRSR2 knockdown cells incorporated 5-bromodeoxyuridine in in vitro labelling assay ( Supplementary Fig. 13b ), indicating that the ZRSR2-deficient cells divide slower than the control cells. We further tested the in vivo tumorigenic potential of ZRSR2 knockdown K562 cells in mice. Cells were injected subcutaneously in NOD-scid-gamma mice and the tumour growth was assessed. ZRSR2-deficient K562 cells produced smaller tumours as compared with the cells transduced with control shRNA ( Fig. 6b ). These results illustrate that downregulation of ZRSR2 suppresses cellular growth both in vitro and in vivo . 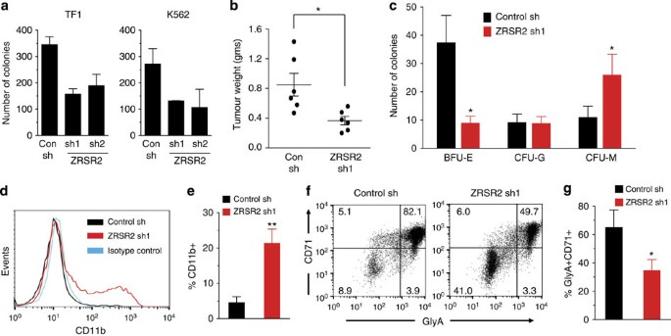Figure 6: Stable knockdown of ZRSR2 alters cell growth and differentiation. (a) Colony-forming ability of TF-1 and K562 cells transduced with ZRSR2 shRNA and control vectors was evaluated using soft-agar colony assay. One thousand and five hundred cells were seeded in each well of a 24-well plate and colonies were enumerated after 2 weeks. Cells were plated in triplicate and the data are the mean±s.e.m. from multiple experiments (TF-1:n=8 for sh1 andn=3 for sh2; K562:n=2). (b) ZRSR2 knockdown and control K562 cells were transplanted into the flank of NOD-scid-gamma (NSG) mice; tumours were dissected after 2 weeks and weighed. Data represent mean±s.e.m. (c) Cord blood-derived CD34+cells were transduced with ZRSR2 shRNA lentivirus and plated in methylcellulose media containing stem cell factor (SCF), interleukin-3 (IL-3), granulocyte colony-stimulating factor (G-CSF), granulocyte macrophage colony-stimulating factor (GM-CSF) and erythropoietin (EPO), as well as 1 μg ml−1puromycin. Burst-forming unit-erythroid (BFU-E), colony-forming unit-granulocyte (CFU-G) and colony-forming unit-macrophage (CFU-M) colonies were counted after 9 days. Data represent the mean±s.e.m. of three experiments. (d–g) CD34+cells were transduced as inc, cultured in liquid media containing SCF, IL-3, GM-CSF and EPO for 2 weeks and analysed using flow cytometry. (d) A representative overlay of histograms showing staining with αCD11b antibody used as a marker of differentiation towards myeloid lineage. (e) Percentage of CD11b+cells obtained afterin vitrodifferentiation of CD34+cells in four experiments are depicted (mean±s.e.m.). (f) Erythroid differentiation was measured using surface expression of Glycophorin A and CD71 antigens in cells cultured for 2 weeks in the presence of cytokines. Representative dot plots for flow cytometric analysis of ZRSR2 knockdown and control cells are shown. Percentage of cells in each quadrant are indicated. (g) Bar graphs represent percentages of GlyA+CD71+cells from three experiments (mean±s.e.m.). *P<0.05, **P<0.01.P-values were calculated using Student’st-test. Figure 6: Stable knockdown of ZRSR2 alters cell growth and differentiation. ( a ) Colony-forming ability of TF-1 and K562 cells transduced with ZRSR2 shRNA and control vectors was evaluated using soft-agar colony assay. One thousand and five hundred cells were seeded in each well of a 24-well plate and colonies were enumerated after 2 weeks. Cells were plated in triplicate and the data are the mean±s.e.m. from multiple experiments (TF-1: n =8 for sh1 and n =3 for sh2; K562: n =2). ( b ) ZRSR2 knockdown and control K562 cells were transplanted into the flank of NOD-scid-gamma (NSG) mice; tumours were dissected after 2 weeks and weighed. Data represent mean±s.e.m. ( c ) Cord blood-derived CD34 + cells were transduced with ZRSR2 shRNA lentivirus and plated in methylcellulose media containing stem cell factor (SCF), interleukin-3 (IL-3), granulocyte colony-stimulating factor (G-CSF), granulocyte macrophage colony-stimulating factor (GM-CSF) and erythropoietin (EPO), as well as 1 μg ml −1 puromycin. Burst-forming unit-erythroid (BFU-E), colony-forming unit-granulocyte (CFU-G) and colony-forming unit-macrophage (CFU-M) colonies were counted after 9 days. Data represent the mean±s.e.m. of three experiments. ( d – g ) CD34 + cells were transduced as in c , cultured in liquid media containing SCF, IL-3, GM-CSF and EPO for 2 weeks and analysed using flow cytometry. ( d ) A representative overlay of histograms showing staining with αCD11b antibody used as a marker of differentiation towards myeloid lineage. ( e ) Percentage of CD11b + cells obtained after in vitro differentiation of CD34 + cells in four experiments are depicted (mean±s.e.m.). ( f ) Erythroid differentiation was measured using surface expression of Glycophorin A and CD71 antigens in cells cultured for 2 weeks in the presence of cytokines. Representative dot plots for flow cytometric analysis of ZRSR2 knockdown and control cells are shown. Percentage of cells in each quadrant are indicated. ( g ) Bar graphs represent percentages of GlyA + CD71 + cells from three experiments (mean±s.e.m.). * P <0.05, ** P <0.01. P -values were calculated using Student’s t -test. Full size image Next, the implications of ZRSR2 deficiency on myeloid differentiation were investigated using an in vitro model of differentiation of human CD34 + haematopoietic stem cells (HSCs). CD34 + cells enriched from cord blood were transduced with either ZRSR2 shRNA or control shRNA lentivirus, and analysed for in vitro clonogenic growth in methylcellulose media. We observed a marked decrease in the number of Burst-forming unit-erythroid (BFU-E) obtained after 9 days. On the other hand, a notable increase in the number of colony-forming unit-macrophage (CFU-M) occurred, while the number of colony-forming unit-granulocyte (CFU-G) was unaffected ( Fig. 6c ). We confirmed an effective knockdown of ZRSR2 in transduced cells using qRT–PCR ( Supplementary Fig. 14 ). Next, we evaluated the differentiation profile of CD34 + cells using flow cytometry. Following transduction with lentivirus, cells were cultured in the presence of cytokines for 2 weeks. A significant increase in the proportion of CD11b + myeloid cells was observed on knockdown of ZRSR2 ( Fig. 6d,e ). Downregulation of ZRSR2 also resulted in a reduced proportion of erythroid precursors co-expressing Glycophorin A and CD71 surface antigens ( Fig. 6f,g ). These results indicate that suppression of ZRSR2 alters erythroid and myeloid differentiation of HSCs, presumably as a result of dysregulated splicing of genes implicated in haematopoiesis. Pathways regulated by mis-spliced genes in ZRSR2 mutant MDS To reveal the enrichment of functionally related genes among the significantly mis-spliced transcripts in ZRSR2 mutant MDS ( Supplementary Data 1,4 and 5 ), Gene Ontology (GO) analyses was performed using the standard enrichment computation method. A significant enrichment was obtained for several pathways ( P <0.05) including mitogen-activated protein kinase (MAPK) signalling, ErbB signalling and for genes associated with chronic myeloid leukemia and AML ( Fig. 7a ). We sought to identify downstream targets of aberrant splicing of ZRSR2, which may contribute to the disease phenotypes. Several genes, which participate in either haematopoietic differentiation or are implicated in myeloid malignancies, were consistently mis-spliced in all ZRSR2 mutant MDS samples ( Fig. 7b ). For instance, members of E2F transcription factors—E2F1, E2F2, E2F3, E2F4 and E2F6—which function during myeloid differentiation [29] , [30] , [31] , [32] , [33] , [34] , [35] , exhibit splicing defects in ZRSR2 mutant cells. Similarly, various regulators of MAPK signalling, including MAPK1, MAPK3, RAS guanyl releasing proteins and RAF serine/threonine protein kinases contain U12-type introns and were mis-spliced in ZRSR2 mutant cells. These proteins mediate vital signalling cascades and their role in maintaining physiological haematopoiesis has been identified [36] , [37] , [38] , [39] , [40] , [41] , [42] , [43] , [44] . Another interesting candidate is the tumour suppressor gene, PTEN , loss of which impairs HSC activity, alters their lineage commitment and leads to myeloid disorders in mice [45] , [46] . Dysregulation of these genes through aberrant splicing can potentially have direct implications on haematopoietic differentiation and may contribute to the pathogenesis of MDS. Further investigations are necessary to identify effector(s) of the MDS phenotype in ZRSR2 mutant cells. 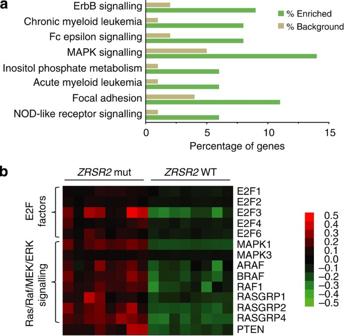Figure 7: GO analyses of mis-spliced genes inZRSR2mutant MDS. (a) GO analysis of 251 significantly mis-spliced genes inZRSR2mutant MDS shows their enrichment in a number of essential biological pathways (P<0.05). (b) Heat map portrays the relative scale of aberrant retention of U12-type introns in genes involved in haematopoietic development. MSI values for U12-type introns inZRSR2mutant and control samples were utilized for depiction of mis-splicing. Figure 7: GO analyses of mis-spliced genes in ZRSR2 mutant MDS. ( a ) GO analysis of 251 significantly mis-spliced genes in ZRSR2 mutant MDS shows their enrichment in a number of essential biological pathways ( P <0.05). ( b ) Heat map portrays the relative scale of aberrant retention of U12-type introns in genes involved in haematopoietic development. MSI values for U12-type introns in ZRSR2 mutant and control samples were utilized for depiction of mis-splicing. Full size image Overall, our results demonstrate that ZRSR2 mutations lead to aberrant splicing, primarily involving U12-type introns. These splicing defects are also corroborated in knockdown cells, which display alterations in growth and differentiation, substantiating an essential and non-redundant role of ZRSR2 in the U12-dependent spliceosome. Discovery of mutations in several spliceosome genes in MDS strongly suggest existence of dysfunctional splicing machinery in this disease. Interestingly, majority of the mutated genes including SF3B1 , U2AF1 , ZRSR2 , SRSF2 , SF1 and SF3A1 (ref. 8 ), encode for components of E/A splicing complex, which is involved in the recognition of splice sites. Recurrent somatic mutations in these genes, which occur mutually exclusively, indicate that the disruption of initial splicing steps is a common feature in MDS. Therefore, these mutations can be predicted to cause widespread alterations in splicing and gene expression. However, contrary to this hypothesis, mutations in U2AF1 and SF3B1 exert splicing changes in a specific subset of introns and exons [11] , [47] , [48] . Hence, this raises the question whether mutations of each splice factor has a distinctive effect on the splicing machinery, which possibly results in diverse phenotypes. In fact, evidence shows an association between splice factor mutation and the clinical phenotype. SF3B1 mutations are found at high frequency in MDS subtypes characterized by the presence of ring sideroblasts, SRSF2 mutations are highly associated with chronic myelomonocytic leukemia, while mutations in ZRSR2 are often observed in RAEB-1 and RAEB-2 subtypes [8] , [13] , [47] , [49] , [50] , [51] , [52] . In this study, we demonstrate that the depletion of ZRSR2 leads to a specific splicing defect by disrupting the splicing of the entire subset of U12-type introns. Therefore, our study and previous reports indicate that the mutations in individual splice factors are likely to alter the function of splicing machinery in an exclusive manner. Our results define an essential role of ZRSR2 in splicing of U12-type introns and propose it as one of the key components of the minor spliceosome. Our lentiviral shRNA-mediated knockdown approach demonstrates a specific defect in splicing of U12-type introns, which can be reversed by transient overexpression of ZRSR2. Most notably, RNA-Seq revealed that the transcriptome of ZRSR2 mutant MDS exhibited several splicing defects, invariably resulting from inefficient splicing of the U12-type introns. Surprisingly, the U2-type introns were spliced with similar efficiency as the control cells. Although ZRSR2 was shown to be required for in vitro splicing of U2-type introns [22] , [23] , our results provide the first evidence that in vivo splicing of U2-type introns is essentially unaffected in the absence of ZRSR2. We detect significant retention of U2-type introns only in transcripts that contain U12-type introns. Rare U2-type introns independent of the U12 transcripts appear in our analysis of mis-spliced introns. However, these introns exhibit weak mis-splicing phenotype and do not indicate any specificity with respect to either splice site strength or intron length, and therefore, are probable outliers in our analysis. These results signify ZRSR2 is crucial to the U12 spliceosome machinery, while it may have either a limited or redundant role in the U2 machinery. In addition, ZRSR2 has been identified as a component of U11/U12 snRNP [53] . The importance of ZRSR2 in U12-dependent spliceosome was also noted by the inability of cell extract lacking ZRSR2 to form a U12 splicing complex assembly in in vitro assays [23] . Further, a perfect correlation exists in the phylogenetic distribution of organisms that have both ZRSR2- and U12-dependent splicing, which also strongly supports the involvement of this splice factor in the U12 machinery [23] . Our computational analysis also demonstrates that ZRSR2 mutations cause mis-splicing of a majority of U12-type introns, except for a minor subset with weaker U12-type splice sites. ZRSR2 contacts the 3′-splice site of the U12-type intron of P120 transcript by binding the A residue of the AC dinucleotide at the 3′-splice site [23] . This suggests that ZRSR2 is needed for recognition of 3′-splice sites in U12-type introns. Interestingly, the U12-spliceosome complexes (Complex A and Complex B/C) failed to assemble at P120 pre-mRNA in its absence [23] , indicating that recognition of the whole intron is impaired. Analysis of our RNA-Seq data also suggests that the ZRSR2-mediated 3′-splice site recognition is required for the 5′-splice site and branch site recognition. This is evident by activation of cryptic 5′-splice site sequences in certain U12-type intron containing transcripts such as DRAM2, TAPT1 and VPRBP in ZRSR2 mutant MDS ( Supplementary Fig. 15 ). Similar instances of cryptic splice sites were previously reported for deficiency of RNPC3 and U11–48K, proteins also involved in the U12 splicing machinery [54] , [55] . The cryptic splice junctions observed in ZRSR2 mutant cells were invariably U2 type. Unlike the U2-dependent spliceosome, the U12-dependent machinery has been less well understood and proteins involved in splice-site recognition are not clearly defined. U12 spliceosome was initially uncovered as a machinery instrumental in excising introns lacking the consensus GT-AG splice site termini [56] . However, it was soon recognized that this splicing complex was responsible for a unique subset of evolutionary conserved introns, which had a highly conserved splice-site recognition sequences distinct from the U2-type introns [16] , [17] , [21] , [24] and which used different snRNPs than those used in U2 machinery [18] , [19] . Although the U12-type introns comprise ~0.5% of all human introns, they exist in several crucial genes involved in vital cellular processes [57] . Germline mutations in the RNU4ATAC gene, which encodes for an essential component of the U12 spliceosome, have been shown to cause MOPD1/TALS (Microcephalic Osteodysplastic Primordial Dwarfism type 1/Taybi–Linder Syndrome), a rare developmental disorder in humans [58] , [59] . Biallelic mutations in the RNPC3 gene, which encodes for a 65-kDa constituent of U11/U12 di-snRNP, also lead to isolated familial growth hormone deficiency [55] . Moreover, an intact U12 spliceosome is essential for the development of Drosophila (despite the presence of <20 U12-type introns in its genome) and zebrafish [60] , [61] , [62] . Thus, the questions raised in the context of myeloid neoplasms are: what are the consequences of the impairment of U12 splicing specifically in HSCs and how the ZRSR2 mutations (and other spliceosome gene mutations, in general) contribute to leukemogenesis. We show that knockdown of ZRSR2 in human HSCs alters their in vitro differentiation potential. Reduced differentiation occurs towards erythroid lineage accompanied by a higher proportion of CD11b + myeloid cells on knockdown of ZRSR2. These results suggest that a competent U12 spliceosome is required for normal myeloid differentiation. Further investigations will focus on identifying downstream target genes, which on mis-splicing lead to pathogenic consequences in MDS. In this study, the GO analysis of U12-type genes identifies few such molecular pathways with potential involvement in the MDS phenotype. We find that genes encoding E2F transcription factors and several components of the Ras/Raf/MEK/ERK signalling exhibit aberrant splicing of U12-type introns consistently in all ZRSR2 mutant MDS. These proteins have been implicated in normal and malignant haematopoiesis and represent possible candidates for future investigations. Studies using murine models will help identify downstream targets and better understand the role of ZRSR2-mediated splicing in haematopoietic differentiation. Pathway analysis of mis-spliced genes also revealed a strong enrichment of key cellular functions such as RNA transport, cell cycle, cellular response to stress, response to DNA damage stimulus, protein transport, protein serine/threonine kinase activity and ribonucleotide binding among the mis-spliced genes ( Supplementary Fig. 16 ). These functional classes have been previously attributed to the genes containing the U12-type introns [57] . Downregulation of ZRSR2 impaired in vitro clonogenic ability and suppressed tumour formation in mice. Overall, the ZRSR2 knockdown leukemia cells showed a general tendency to grow slower than the control cells. This observation is similar to the effect on cell growth reported for other spliceosome mutations. Expression of mutant U2AF1 suppressed the growth of cell lines and resulted in lower reconstitution potential in mice [8] . Cell cycle arrest and inhibition of growth in leukemia cell lines is also attributed to downregulation of SF3B1 (ref. 63 ). Therefore, the spliceosome mutations do not seem to contribute towards a proliferative advantage of the haematopoietic precursors in MDS. How these cells harbouring spliceosome mutations achieve clonal expansion remains unclear. One explanation can be that other accompanying genetic alterations are necessary to confer a proliferative advantage. In fact, mutations in several components of epigenetic machinery co-occur with spliceosome mutations. A high incidence of co-occurrence of mutations in the TET2 and ZRSR2 genes has been noted in MDS [8] , [13] . Loss of TET2 has been shown to lead to myeloproliferation and transformation of haematopoietic precursors in mice [64] , [65] . Therefore, mutations in TET2 are likely to promote clonal dominance. Mutations in spliceosome genes, which occur early during leukemogenesis [66] , might play a prominent role in modifying the differentiation potential of myeloid precursors, thus contributing to abnormal precursor phenotype, which is a hallmark of MDS. Further studies into co-operativity between mutations in spliceosome and epigenetic modifier genes in pathogenesis of myeloid disorders are therefore warranted. Generation of stable ZRSR2 knockdown cell lines Lentiviral shRNA vectors (pLKO.1) were either purchased from Sigma or assembled by cloning the shRNA hairpin loop sequence into the AgeI/EcoRI sites of the empty vector. The target sequence for the ZRSR2 shRNAs sh1 and sh2 are 5′-CAACAGTTCCTAGACTTCTAT-3′ and 5′-AGCAGCCCTTTCTCTGTTTAA-3′, respectively. MISSION pLKO.1-puro Non-Mammalian shRNA Control (SHC002; Sigma) was used as control vector for transduction. To generate lentiviral particles, 293T cells (kindly provided by Dr Bing Lim, Genome Institute of Singapore, Singapore) were co-transfected with shRNA plasmid and the packaging plasmids, pMISSIONgagpol and pMISSIONvsvg (Sigma) using Lipofectamine 2000 (Invitrogen). Virus containing supernatant was collected after 48 and 72 h, filtered through 0.45 μm filter and stored in aliquots at −80 °C. TF-1 and K562 cells (American Type Culture Collection) were infected with lentivirus for two rounds, 24 h apart, in the presence of 5 μg ml −1 protamine sulfate. Transduced cells were selected in puromycin to generate stable knockdown cell lines. The knockdown was verified using qPCR and western blotting. Western blot analysis Total protein lysates were prepared using M-PER Mammalian Protein Extraction Reagent (Thermo Scientific) containing protease inhibitor cocktail (Roche). Twenty-five micrograms of protein was resolved on 10% SDS–PAGE gel and transferred to Immobilon-P polyvinylidene difluoride membrane (Millipore). Anti-ZRSR2 antibody (1:2,500 dilution; kindly provided by Dr Michael Green, University of Massachusetts Medical School, MA) was used to determine ZRSR2 protein expression. The membrane was stripped before probing with anti-GAPDH antibody (1:5,000 dilution; Cell Signaling Technology). Minigene splicing assays P120 reporter construct was generously provided by Dr Richard A. Padgett, Cleveland Clinic, Cleveland, OH, and the GH1 minigene plasmid was provided by Dr Kinji Ohno, Center for Neurological Diseases and Cancer, Nagoya, Japan. 293T cells were transfected with P120 or GH1 plasmids using jetPRIME transfection reagent (Polyplus Transfection SA). Briefly, cells in 60 mm dish were transfected with 200 ng of reporter plasmid. Cells were harvested 48 h after transfection and total RNA was extracted using AxyPrep Multisource Total RNA Miniprep Kit (Axygen). RNA was treated with DNase I followed by complementary DNA synthesis using RevertAid First Strand cDNA Synthesis Kit (Thermo Scientific). For P120 minigene assay, plasmid-specific primer was used for reverse transcription. The cDNA was used as a template to amplify the region of P120 gene containing intron F at 94 °C for 2 min followed by 25 cycles of 94 °C for 30 s, 60 °C for 40 s, 72 °C for 40 s and a final extension at 72 °C for 7 min. Amplified PCR product was resolved on agarose gel, stained with ethidium bromide and photographed. Bands corresponding to spliced (112 bp) and unspliced (211 bp) products were quantified using Image Lab software (Biorad). For GH1 minigene, reverse transcription was performed using random primers. The PCR to amplify the GH1 transcript was performed at 94 °C for 2 min followed by 28 cycles of 94 °C for 30 s, 60 °C for 40 s, 72 °C for 40 s and a final extension at 72 °C for 7 min. Amplicons corresponding to fully spliced and exon skipped transcripts measured 447 and 327 bp, respectively. The sequences of primers used for RT–PCR are provided in the Supplementary Table 1 . RT–PCR to determine splicing efficiency of U2-type and U12-type introns Splicing of U2-type and U12-type introns was measured using qRT–PCR [47] , [59] . Briefly, RNA was treated with DNase I (Thermo Scientific) followed by reverse transcription using RevertAid M-MuLV Reverse Transcriptase (RevertAid First Strand cDNA Synthesis Kit, Thermo Scientific) in the presence of random primers. Spliced and unspliced levels of introns were measured using two separate qPCRs and normalized to GAPDH transcript levels. PCR conditions included an initial denaturation at 95 °C followed by 40–50 cycles of denaturation at 95 °C for 15 s and annealing/extension at 60 °C for 30 s. Primer sequences used for U2-type and U12-type introns are provided in Supplementary Table 1 . Splicing efficiency was calculated as a ratio of relative quantities of spliced and unspliced pre-mRNA levels and was set as 1 for the control transduced cells. Overexpression of ZRSR2 Full-length coding sequence of human ZRSR2 gene (1449, bp) was amplified using PCR and cloned into BamHI/NotI sites of pCDNA3.1 expression vector (Invitrogen). Two micrograms of plasmid was used to transfect 293T cells in a 60-mm petri dish using jetPRIME transfection reagent (Polyplus Transfection), according to the manufacturer’s protocol. RNA was extracted 72 h after transfection and overexpression of ZRSR2 was verified using qPCR. RT–PCR to assess the splicing efficiency of U12-type introns was performed as described above. Bone marrow samples Bone marrow aspirates of diagnostic samples, including MDS and non-malignant cases, were obtained at the MLL Munich Leukemia Laboratory. Informed consent was obtained in accordance with the Declaration of Helsinki and approved by the Institutional Review Board of the MLL. Unfractionated bone marrow mononuclear cells were lysed and total RNA was extracted using RNeasy Kit (Qiagen). Soft-agar colony assay Colony-forming ability of TF-1 and K562 cells was determined by plating the cells in semi-solid media containing agar. The bottom layer consisted of 0.5% agar supplemented with 20% fetal bovine serum, RPMI-1640 medium and antibiotics/antimycotic (Gibco). One thousand and five hundred cells were mixed with the top agar layer, which contained 0.35% agar and RPMI-1640 medium, fetal bovine serum, L -glutamine, β-mercaptoethanol and antibiotics/antimycotic, which was plated in each well of 24-well dish. Two weeks after plating, colonies were enumerated under the microscope from triplicate wells. Xenograft tumour model All mice experiments were approved by the Institutional Animal Care and Use Committee, National University of Singapore, Singapore. Ten million K562 cells were resuspended in 50% matrigel and injected subcutaneously into flank of 8-week-old female NOD-scid-gamma mice. Each mouse was injected with control cells in one flank and the ZRSR2 knockdown cells in the other. Once tumours were palpable, mice were killed, tumours were harvested and weighed. In vitro differentiation of human CD34 + cells CD34 + cells were enriched from fresh cord blood and transduced twice, 24 h apart, with ZRSR2 shRNA lentivirus. For colony assay, 2,500 transduced cells were plated per well in a six-well dish in methylcellulose media (Stemcell Technologies) supplemented with stem cell factor, granulocyte colony-stimulating factor, granulocyte macrophage colony-stimulating factor, interleukin-3 and erythropoietin, and containing puromycin. Colonies were enumerated after 9 days. In some experiments, cells were harvested from colonies and used to extract RNA. Downregulation of ZRSR2 was examined using qRT–PCR. For liquid culture, cells were maintained in the presence of single cell factor, granulocyte macrophage colony-stimulating factor, interleukin-3, erythropoietin and puromycin for 2 weeks. Expression of Glycophorin A and CD71 (erythroid lineage) and CD11b (myeloid lineage) was determined using flow cytometry. Data were analysed using Flowjo software. RNA sequencing Library preparation and sequencing . cDNA libraries were prepared using TruSeq RNA Sample Preparation Kit (Illumina), according to the manufacturer’s protocol. One microgram of total RNA was used for library preparation and paired-end adapters were ligated to DNA fragments before amplification and sequencing on a HiSeq 2000 instrument (Illumina) with 100 bp paired-end reads, according to manufacturer’s protocol. We first mapped the sequenced reads to the reference transcript in the database obtained from RefSeq, Ensemble and UCSC known genes using bowtie, and unmapped or poorly mapped reads were realigned to human reference genome (hg19) with the Blat software. This two-step mapping procedure is included in genomon-fusion ( http://genomon.hgc.jp/rna/ ) pipeline. The mapped reads were organized into five different libraries as follows: (a) exon read library, (b) intron read library, (c) exon–intron junction read library, (d) exon–exon junction read library and (e) intergenic read library. The gene classification was done using all known RefSeq transcripts. To be considered as a real junction, two criteria were applied. First, we required the splice junction to be supported by at least five reads and aligned reads spanned a minimal of 4 bp on each side of the junction. Differential splicing analysis . To identify splicing events, we introduced a parameter called MSI, which is equivalent to Percent Spliced-in values used for alternative splicing analysis [67] , [68] and modified to cater to different splicing events such as intron retention, exon skip and incorrect splice site usage (see Supplementary Fig. 5 for mathematical expression of MSI). For identification of differential splicing between two samples, the difference in MSI (ΔMSI) was applied: ΔMSI=MSI ZRSR2 mutant −MSI control . Furthermore, we used the Fisher’s exact test to evaluate the significance of such difference and adjusted P -value by FDR analysis to minimize the false positives. For identification of differentially spliced events among two genotypes, we performed all possible pairwise analyses between ZRSR2 mutant MDS and control ( ZRSR2 WT MDS and normal BM) samples. These include 32 comparisons each between ‘ ZRSR2 mutant MDS’ and ‘ ZRSR2 WT MDS’ or ‘ ZRSR2 mutant MDS’, and ‘normal BM’ (total 64 pairwise comparisons). As control, ZRSR2 WT MDS samples were compared with normal BM samples (4 × 4=16 comparisons). A similar approach was used to compare the mis-splicing in ZRSR2 knockdown versus control-transduced TF-1 cells. Statistical difference of P ≤0.01 and difference in ΔMSI >20 were considered as significant differential splicing in each comparison. To identify an overall significant mis-splicing between the two genotypes ( ZRSR2 mutant versus controls), we considered the frequency of occurrence of mis-splicing events in pairwise comparisons and applied an FDR of ≤0.01 for intron retention and ≤0.02 for abnormal splice site recognition and exon skip analysis, using the control-versus-control comparisons as background. For intron retention analysis, we selected events where at least one read overlaps an intron and flanking exons at each of the two junctions, and the total number of such junction read counts was a minimum of 4, in at least one sample. We also applied the criteria that ≥95% of the intron was covered by at least one read ( Supplementary Fig. 17 ). Classification of introns . First, position weight matrices were generated based on the 5′- and 3′-splice sites and the branch site sequence. These matrices were used to scan the introns of interest and the introns were then categorized as U2-type or U12-type based on the mapping score [27] . Gene expression analysis . The relative abundance of transcripts was quantified using normalized fragments per kilobase of transcript per million fragments mapped, which were calculated using bedtools with a transcriptome reference. Gene function analysis for mis-spliced genes . Genes significantly mis-spliced in ZRSR2 mutant MDS cases were analysed using GO tools, to identify enriched GO terms for biological pathways, biological processes and molecular functions. Significant enrichment was computed based on the Fishers’ exact test, using the numbers of mis-spliced genes compared with the numbers in the genome for each GO term. The obtained P -value was further corrected for FDR as described [69] . GO pathway analysis tool used was the MetaCore from GeneGO ( https://portal.genego.com/ ) and the GO analysis for biological processes and molecular functions was done with DAVID ( http://david.abcc.ncifcrf.gov ). The corrected P -value cutoff of 0.05 was used for significant enriched GO terms. Heat maps were created for enriched biological processes and molecular functions, using Cluster 3.0 software. Validation of mis-spliced genes . Intron retention in ZRSR2 mutant MDS was verified using qRT–PCR [70] . Expression of each intron was normalized against the expression of flanking exons. For validation of other mis-spliced introns, qPCR or conventional PCR were used. GAPDH was used as the normalization control for cDNA input. Primer sequences are available in the Supplementary Table 1 . How to cite this article: Madan, V. et al. Aberrant splicing of U12-type introns is the hallmark of ZRSR2 mutant myelodysplastic syndrome. Nat. Commun. 6:6042 doi: 10.1038/ncomms7042 (2015). Accession codes: The RNA-Seq data have been deposited in the NCBI Gene Expression Omnibus under accession code GSE63816 .